Cell–cell adhesion genesCTNNA2andCTNNA3are tumour suppressors frequently mutated in laryngeal carcinomas Laryngeal squamous cell carcinoma is a frequent and significant cause of morbidity and mortality. Here we explore the biological basis of this aggressive tumour, and identify two cell–cell adhesion genes as recurrently mutated in this malignancy. We first perform exome sequencing of four laryngeal carcinomas and their matched normal tissues. Among the 569 genes found to present somatic mutations, and based on their recurrence or functional relevance in cancer, we select 40 for further validation in 86 additional laryngeal carcinomas. We detect frequent mutations (14 of 90, 15%) in CTNNA2 and CTNNA3 -encoding α-catenins. Functional studies reveal an increase in the migration and invasive ability of head and neck squamous cell carcinoma cells producing mutated forms of CTNNA2 and CTNNA3 or in cells where both α-catenins are silenced. Analysis of the clinical relevance of these mutations demonstrates that they are associated with poor prognosis. We conclude that CTNNA2 and CTNNA3 are tumour suppressor genes frequently mutated in laryngeal carcinomas. Head and neck carcinomas are an anatomically diverse and molecularly heterogeneous group of malignancies involving the oral cavity and oropharynx, nasopharynx, hypopharynx, larynx, ear, nasal cavity and paranasal sinuses, as well as the thyroid, parathyroid and salivary glands. Head and neck squamous cell carcinoma (HNSCC) represents >90% of all head and neck cancers and arises from the mucosa of the upper aerodigestive tract. With a worldwide incidence exceeding half a million cases annually, HNSCC poses a major health risk and is one of the leading causes of mortality in developing nations [1] . The most significant risk factors to develop HNSCC remain tobacco and alcohol abuse. It is now well established that HNSCC is a heterogeneous disease, both at the molecular and clinical level, which arises from a multistage pathogenesis process [2] . Despite advances in the clinical classification of the disease, a global genomic perspective is still needed to shed light on the whole mutational landscape and underlying molecular mechanisms characteristic of this type of tumour. In this regard, recent works of whole-exome sequencing of HNSCC have been published [3] , [4] . In addition to identifying genes previously known to be involved in HNSCC, such as TP53 , CDKN2A , PTEN , PIK3CA and HRAS , these studies have proposed NOTCH1 as a possible key tumour suppressor gene in the HNSCC carcinogenic process. Other genes such as IRF6 , TP63 and FBXW7 have also been described in these reports as important HNSCC-mutated genes. However, these next-generation sequencing HNSCC studies did not identify novel cancer-related genes. Here we report the characterization of the mutational landscape of four laryngeal squamous cell carcinomas, with a validation set of 86 additional cases. To our knowledge, this is the first high-throughput genomic study on a large cohort of biologically homogeneous laryngeal squamous cell carcinoma samples surgically isolated from patients who had not received chemotherapy or radiotherapy before surgery. This approach circumvents the noise derived from the biological and clinical heterogeneity that hindered previous studies on HNSCC in which laryngeal carcinomas were only minimally represented. This strategy has allowed us to unveil frequent somatic mutations targeting cell–cell adhesion genes CTNNA2 and CTNNA3 in larynx cancer. In this work, we also provide functional analyses demonstrating that cells expressing mutated versions of CTNNA2 and CTNNA3 exhibit enhanced migration and invasion capabilities, a behaviour recapitulated by HNSCC cells in which expression of these α-catenins was silenced. Finally, we perform clinical analyses that show a poor prognosis in patients with CTNNA2 or CTNNA3 mutations. CTNNA2 and CTNNA3 mutations in larynx cancer To better understand the molecular pathogenesis of HNSCC and to minimize the known biological and molecular heterogeneity among tumours originated from different head and neck anatomical locations such as the oral cavity, pharynx, larynx and paranasal sinuses [5] , [6] , we have carried out a mutational analysis of laryngeal carcinomas. 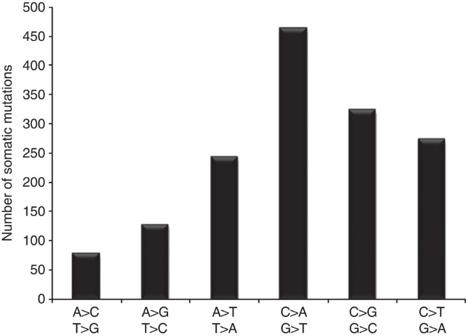Figure 1: Mutational profile of whole-exome-sequenced samples from patients with laryngeal carcinoma. Each mutation type is expressed as reference base >mutated base in either strand. The number in each group is the aggregate of all four exomes. To this purpose, we first performed whole-exome sequencing of matched tumour and normal samples from four individuals with laryngeal squamous cell carcinoma and a clinical history of tobacco and alcohol abuse ( Table 1 ). The tumour biopsies were taken during the surgical procedure and none of the patients had received chemotherapy or radiotherapy before surgery. We achieved 106-fold mean sequence coverage of targeted exonic regions. On average, 89% of the exome positions were covered by more than eight reads with Phred quality higher than 30 (callable exome; Supplementary Table S1 ). We identified a median of 260 somatic mutations per case, which represents about seven mutations per megabase of sequenced DNA ( Supplementary Data 1 ). This mutational rate agrees with data recently reported for head and neck carcinomas from different locations [3] , [4] as well as for other smoking-related malignancies [7] . The most common substitution found in these laryngeal carcinomas was G>T/C>A ( Fig. 1 ), which is also consistent with data from studies on other smoking-related tumours [7] . Analysis of the identified somatic mutations predicted that 606 of them result in protein-coding changes in 569 genes ( Supplementary Data 2 ). To determine whether any of these genes was recurrently mutated, we next analysed a validation set of 86 laryngeal squamous cell carcinomas from patients who had not received chemotherapy or radiotherapy before surgery. To avoid any putative mutational bias derived from heterogeneity among HNSCCs from different sites [5] , [6] , we carefully selected patients whose tumours were unequivocally diagnosed as laryngeal squamous cell carcinomas ( Supplementary Data 3 ). To perform the validation analysis, we focused on 40 genes mutated in more than one of the four exome-sequenced tumours or whose biological function was presumed to be relevant for cancer development ( Supplementary Data 4 ). Then, we used Somatic Mutation Identification in Pooled Samples (SMIPS), a pooled sequencing strategy with the ability to identify recurrent mutations, as assessed in previous genomic studies of chronic lymphocytic leukaemia [8] , [9] , [10] . Analysis of this additional set of 86 laryngeal carcinomas led us to identify CTNNA2 and CTNNA3 , encoding cell–cell adhesion α-catenins [11] , [12] , as novel recurrently mutated genes in this aggressive malignancy ( Fig. 2a ). 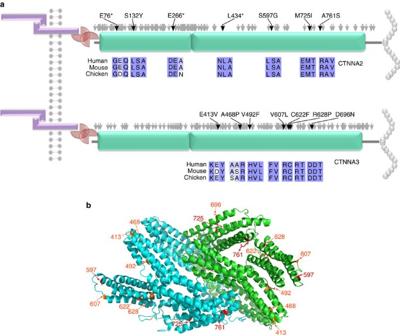Figure 2:CTNNA2andCTNNA3mutations identified in laryngeal carcinomas. (a) Schematic representation of the human CTNNA2 and CTNNA3 adhesion proteins with different somatic alterations found in larynx cancer samples (black) and COSMIC (grey). Green blocks identify the two vinculin-like domains in each α-catenin. CTNNA2 and CTNNA3 are depicted bound to cadherin (violet rectangles) through β-catenin (red arcs), and to actin filaments (grey circles). (b) Structural localization of CTNNA2 and CTNNA3 mutations. The residues corresponding to mutations in CTNNA2 (red) and CTNNA3 (orange) are shown over the structure of a CTNNA1 dimer (pdb id. 4IGG). We found seven tumours with mutations in CTNNA2 and six tumours with mutations in CTNNA3 , including one case harbouring two different missense mutations in this latter gene ( Table 2 ). These cell–cell adhesion genes were among the most frequently mutated genes (15% when considered together) in our patient series. Table 1 Biological characteristics of HNSCC samples analysed by whole-exome sequencing. Full size table Figure 1: Mutational profile of whole-exome-sequenced samples from patients with laryngeal carcinoma. Each mutation type is expressed as reference base >mutated base in either strand. The number in each group is the aggregate of all four exomes. Full size image Figure 2: CTNNA2 and CTNNA3 mutations identified in laryngeal carcinomas. ( a ) Schematic representation of the human CTNNA2 and CTNNA3 adhesion proteins with different somatic alterations found in larynx cancer samples (black) and COSMIC (grey). Green blocks identify the two vinculin-like domains in each α-catenin. CTNNA2 and CTNNA3 are depicted bound to cadherin (violet rectangles) through β-catenin (red arcs), and to actin filaments (grey circles). ( b ) Structural localization of CTNNA2 and CTNNA3 mutations. The residues corresponding to mutations in CTNNA2 (red) and CTNNA3 (orange) are shown over the structure of a CTNNA1 dimer (pdb id. 4IGG). Full size image Table 2 Somatic mutations affecting CTNNA2 and CTNNA3 in the validation series. Full size table Analysis of the mutational spectrum in both α-catenin genes is consistent with the hypothesis that CTNNA2 and CTNNA3 might act as tumour suppressor genes ( Fig. 2a ). Thus, 13 of the identified mutations were predicted to be deleterious to the encoded protein through 10 missense mutations of the vinculin-like domains, with a further 3 truncating the protein through the introduction of premature stop codons ( Table 2 ). Further, no obvious clustering of mutations was observed when the structure of the vinculin domains was taken into account ( Fig. 2b ). Exploration of the COSMIC database [13] revealed that mutations in both α-catenin genes have been annotated in different malignancies ( Fig. 2a ), whereas some CTNNA3 mutations have been recently found in non-small cell lung carcinomas [14] . Further, a very recent analysis of the cbioportal database [15] has revealed the annotation of many CTNNA2 and CTNNA3 mutations in a spectrum of different malignancies, whereas the Cancer Cell Line Encyclopedia [16] has annotated 83 and 19 different cancerous cell lines with mutations in CTNNA2 and CTNNA3, respectively. Collectively, these data reinforce that CTNNA2 and CTNNA3 mutations are present in numerous cancer types and expand the oncological interest of these α-catenin genes beyond laryngeal carcinomas. CTNNA2 and CTNNA3 mutations increase cell invasion CTNNA2 and CTNNA3 are key proteins of the adherens junctional complex in epithelial cells and have a crucial role in cellular adherence [11] , [12] , [17] , [18] . To investigate the functional relevance of CTNNA2 and CTNNA3 in HNSCC cells, we performed both RNA interference and complementary DNA overexpression studies of both genes and interrogated key biological processes for tumour progression. We first carried out a cell adhesion profile assay, which revealed that silencing and overexpression of CTNNA2 and CTNNA3 mainly affected laminin-dependent adhesion of HNSCC cells SCC-2 ( Fig. 3a ) and SCC-40 ( Fig. 4a and Supplementary Fig. S1 ). Subsequently, we analysed by time-lapse microscopy the capacity of these cells to migrate through a scratch wound in laminin-coated plates. These experiments revealed that CTNNA2 and CTNNA3 silencing confers SCC-2 cells ( Fig. 3b , Supplementary Movies 1 and 2 ) and SCC-40 cells ( Fig. 4b ) an enhanced ability to migrate through the wound compared with control cells. 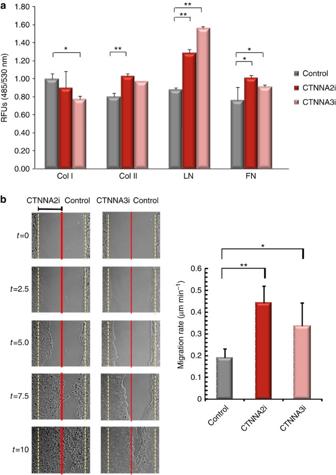Figure 3: Adhesion profile and migration of SCC-2 cells after silencing or overexpression ofCTNNA2andCTNNA3. (a) Following CTNNA2 and CTNNA3 silencing, binding capacity of SCC-2 on different extracellular matrix components was assessed. Affinity is expressed as relative fluorescence units (RFU). ‘i’ refers toCTNNA2orCTNNA3silenced cells, and ‘o’ to cells overexpressingCTNNA2orCTNNA3. Col I, type-I collagen; Col II, type-II collagen; FN, fibronectin; LN, laminin. Statistical analyses were performed by Student’st-test with *P<0.05 and **P<0.01. Error bars represent mean±s.e.m. of three biological replicates. (b) Distance covered by the migration edge from the initial site was measured at different times and graphically represented. Pictures at different times from a representative assay are shown. Statistical analyses were performed by Student’st-test with *P<0.05 and **P<0.01. Error bars represent mean±s.e.m. of three to five biological replicates. Scale bars, 250 μm. Figure 3: Adhesion profile and migration of SCC-2 cells after silencing or overexpression of CTNNA2 and CTNNA3 . ( a ) Following CTNNA2 and CTNNA3 silencing, binding capacity of SCC-2 on different extracellular matrix components was assessed. Affinity is expressed as relative fluorescence units (RFU). ‘i’ refers to CTNNA2 or CTNNA3 silenced cells, and ‘o’ to cells overexpressing CTNNA2 or CTNNA3 . Col I, type-I collagen; Col II, type-II collagen; FN, fibronectin; LN, laminin. Statistical analyses were performed by Student’s t -test with * P <0.05 and ** P <0.01. Error bars represent mean±s.e.m. of three biological replicates. ( b ) Distance covered by the migration edge from the initial site was measured at different times and graphically represented. Pictures at different times from a representative assay are shown. Statistical analyses were performed by Student’s t -test with * P <0.05 and ** P <0.01. Error bars represent mean±s.e.m. of three to five biological replicates. Scale bars, 250 μm. 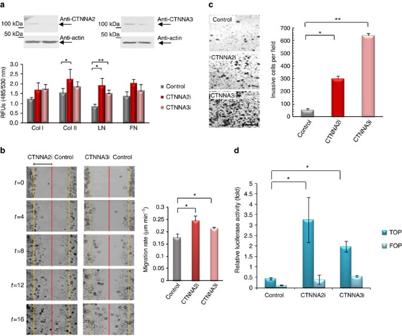Figure 4: Cellular features and β-catenin transcriptional activity of SCC-40 cells after silencing ofCTNNA2andCTNNA3. (a) FollowingCTNNA2andCTNNA3silencing (top), binding capacity of SCC-40 on different extracellular matrix components was assessed (bottom). Col I, type-I collagen; Col II, type-II collagen; FN, fibronectin; LN, laminin. Affinity is expressed as relative fluorescence units (RFU). (b) Distance covered by the migration edge from the initial site was measured at different times and graphically represented. Migration pictures at different times from a representative experiment are shown. (c)CTNNA2andCTNNA3silencing increased invasive capacity of SCC-40 cells. Number of invasive cells were counted and graphically represented. (d) β-catenin transcriptional activity in SCC-40 cells followingCTNNA2andCTNNA3interference. TOP, reporter with optimal Tcf-binding site; FOP, background assessed with Far-from-optimal Tcf-binding site. Statistical analyses were performed by Student’st-test with *P<0.05 and **P<0.01. Error bars represent mean±s.e.m. of three biological replicates. Scale bars, 250 μm and 50 μm inbandc, respectively. Full size image Figure 4: Cellular features and β-catenin transcriptional activity of SCC-40 cells after silencing of CTNNA2 and CTNNA3 . ( a ) Following CTNNA2 and CTNNA3 silencing (top), binding capacity of SCC-40 on different extracellular matrix components was assessed (bottom). Col I, type-I collagen; Col II, type-II collagen; FN, fibronectin; LN, laminin. Affinity is expressed as relative fluorescence units (RFU). ( b ) Distance covered by the migration edge from the initial site was measured at different times and graphically represented. Migration pictures at different times from a representative experiment are shown. ( c ) CTNNA2 and CTNNA3 silencing increased invasive capacity of SCC-40 cells. Number of invasive cells were counted and graphically represented. ( d ) β-catenin transcriptional activity in SCC-40 cells following CTNNA2 and CTNNA3 interference. TOP, reporter with optimal Tcf-binding site; FOP, background assessed with Far-from-optimal Tcf-binding site. Statistical analyses were performed by Student’s t -test with * P <0.05 and ** P <0.01. Error bars represent mean±s.e.m. of three biological replicates. Scale bars, 250 μm and 50 μm in b and c , respectively. Full size image We next evaluated the invasive capacity of HNSCC cells under conditions of loss- or gain-of-function of these α-catenins. We found that CTNNA2- and CTNNA3 -silenced clones showed enhanced ability to invade a Matrigel matrix, whereas cells overexpressing these α-catenin genes exhibited a considerably reduced invasive ability ( Figs 4c and 5 ). To gain further insight into the role of the mutations identified in CTNNA2 and CTNNA3 , we performed site-directed mutagenesis experiments on some selected residues of both α-catenin genes. SCC-2 cells overexpressing CTNNA2-S132Y, CTNNA2-E266*, CTNNA3-C622F or CTNNA3-R628P showed significantly enhanced ability to invade a Matrigel matrix when compared with cells overexpressing wild-type CTNNA2 or CTNNA3 cDNA, and had similar phenotype to the parental controls ( Fig. 5 ). Collectively, these results are consistent with the hypothesis that CTNNA2 and CTNNA3 are tumour suppressor genes, whose genetic inactivation endows HNSCC cells with migration and invasion advantages, which may contribute to the progression of larynx cancer. 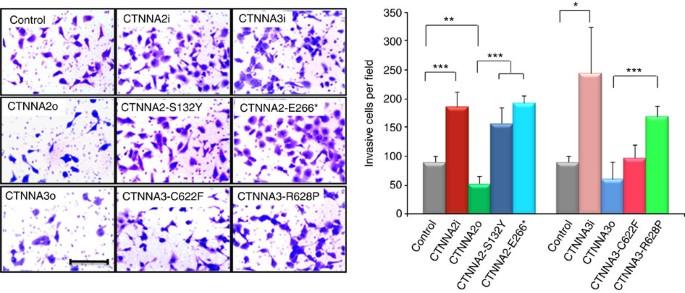Figure 5: Invasive capacity of SCC-2 cells with loss- or gain-of-function ofCTNNA2andCTNNA3. Left, representative microscopic (× 10 magnification) pictures of invasive cells after silencing (i), overexpression of wild-type (o) or overexpression of mutant forms ofCTNNA2andCTNNA3. Right, number of invasive cells for each cell line. Statistical analyses were performed by Student’st-test with *P<0.05, **P<0.01 and ***P<0.005. Error bars represent mean±s.e.m. of three to five biological replicates. Scale bars, 50 μm. Figure 5: Invasive capacity of SCC-2 cells with loss- or gain-of-function of CTNNA2 and CTNNA3 . Left, representative microscopic (× 10 magnification) pictures of invasive cells after silencing (i), overexpression of wild-type (o) or overexpression of mutant forms of CTNNA2 and CTNNA3 . Right, number of invasive cells for each cell line. Statistical analyses were performed by Student’s t -test with * P <0.05, ** P <0.01 and *** P <0.005. Error bars represent mean±s.e.m. of three to five biological replicates. Scale bars, 50 μm. Full size image CTNNA2 and CTNNA3 silencing alters β-catenin signalling To further explore the molecular mechanisms underlying the observed alterations caused by CTNNA2 and CTNNA3 mutations, we next investigated how changes in these genes affect relevant biochemical pathways involving cell–cell adhesion. As these α-catenins interact with β-catenin [11] , [12] , we examined the phosphorylation status of this downstream component of the Wnt pathway, which is altered in many types of cancer [19] , [20] . We found that overexpression of CTNNA2 and CTNNA3 in HNSCC SCC-2 cells grown on laminin caused a substantial decrease in phosphorylation levels of β-catenin at Ser552 ( Supplementary Fig. S2 ). Conversely, silencing of CTNNA2 and CTNNA3 and overexpression of CTNNA2-S132A, CTNNA2-E266* and CTNNA3-R628P in HNSCC cells increased phosphorylation levels of this β-catenin residue ( Supplementary Fig. S2 ). Phosphorylation levels of β-catenin at other Ser and Thr residues did not significantly change after overexpression or silencing of CTNNA2 and CTNNA3 ( Supplementary Fig. S2 ). Phosphorylation of β-catenin at Ser552 results in its translocation from cell–cell contacts into the nucleus [21] , and once β-catenin is translocated, it activates transcription factors of the TCF/LEF-1 family [22] . Therefore, we performed TCF/LEF-1 luciferase reporter assays to evaluate the putative changes in the activity of these transcription factors caused by CTNNA2 and CTNNA3 mutations in laryngeal carcinomas. Silencing of CTNNA2 and CTNNA3 in SCC-2 and SCC-40 cells led to a significant increase of TCF/LEF-1 transcriptional activity when compared with control cells ( Figs 4d and 6 ). In contrast, upregulation of CTNNA2 and CTNNA3 in HNSCC SCC-2 cells was associated with reduced luciferase activity ( Fig. 6 ). Similarly, overexpression of S132A and E266* CTNNA2 mutants as well as that of C622F and R628P CTNNA3 mutants in these cells increased the TCF/LEF-1 transcriptional activity compared with cells overexpressing wild-type genes ( Fig. 6 ). Thus, downregulation of CTNNA2 and CTNNA3 increases phosphorylation of β-catenin at Ser552, which might cause its dissociation from cell–cell contacts, removing the tightly regulated transcriptional control of genes that inhibit cellular motility and invasion, and finally favouring tumour progression. 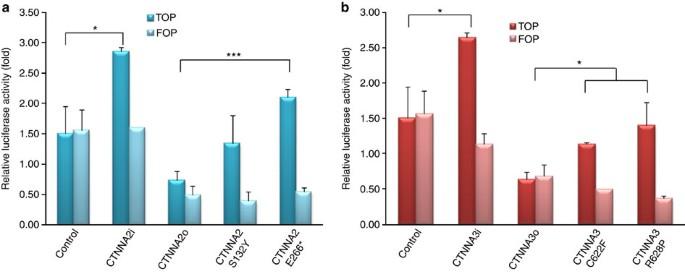Figure 6: β-catenin activity in SCC-2 cells with loss- or gain-of-function ofCTNNA2andCTNNA3. β-catenin transcriptional activity in SCC-2 cells after silencing (i) or overexpression (o) ofCTNNA2(a) andCTNNA3(b). TOP, reporter with optimal Tcf-binding site; FOP, background assessed with Far-from-optimal Tcf-binding site. Statistical analyses were performed by Student’st-test with *P<0.05 and ***P<0.005. Error bars represent mean±s.e.m. of three biological replicates. Figure 6: β-catenin activity in SCC-2 cells with loss- or gain-of-function of CTNNA2 and CTNNA3 . β-catenin transcriptional activity in SCC-2 cells after silencing (i) or overexpression (o) of CTNNA2 ( a ) and CTNNA3 ( b ). TOP, reporter with optimal Tcf-binding site; FOP, background assessed with Far-from-optimal Tcf-binding site. Statistical analyses were performed by Student’s t -test with * P <0.05 and *** P <0.005. Error bars represent mean±s.e.m. of three biological replicates. Full size image CTNNA2 and CTNNA3 mutations are associated with poor prognosis To evaluate the impact of CTNNA2 and CTNNA3 mutations in the clinical outcome of larynx cancer patients, we examined the available clinical data of 86 patients from the validation series, including 7 with mutations in CTNNA2 and/or CTNNA3 ( Supplementary Data 3 ). Then, we constructed a multivariate Cox proportional hazards model including the tumour node metastasis classification of each tumour as a co-variable. This analysis showed that patients in a given stage are four times more likely to die if they have tumours with CTNNA2 or CTNNA3 mutations (hazard ratio: 4.209; 95% confidence interval, 1.045–16.949; P =0.027, log-rank test), which suggests that mutations in these genes are associated with worse clinical prognosis. HNSCC is an aggressive cancer that arises from the epithelial mucosa of the upper aerodigestive track. In recent years, many research projects have tried to gain a comprehensive view of this disease, including two recent works describing for the first time the heterogeneous genomic landscape of HNSCC [3] , [4] . However, survival of these patients has not improved during the last decade, nor has any novel candidate gene related to the progression of this disease been identified in the intervening years. We decided to investigate two factors that may contribute to these disappointing results, namely, the low level of mutational recurrence affecting some genes that drive cancer progression and the anatomical and molecular heterogeneity of HNSCC. Accordingly, this work has focused on the identification and functional analysis of new genes recurrently mutated in a homogeneous cohort of patients suffering from laryngeal squamous cell carcinoma. To identify novel candidate drivers of laryngeal cancer progression, we first analysed the genomes of four tumours compared with the constitutive genome of each patient. A literature-guided examination of the results of this analysis led us to select 40 genes as potentially interesting novel candidates whose mutation might drive the progression of this tumour. We then used SMIPS, a pooled sequencing strategy, to determine which of these genes were indeed recurrently mutated in an extended cohort of 86 patients. This allowed us to identify the α-catenins CTNNA2 and CTNNA3 as new putative drivers of laryngeal carcinoma. Thus, these α-catenins were found altered in ~15% of all the larynx cancer cases, with a uniform distribution amongst glottic and supraglottic tumours. In excellent support of our findings, data mining of the whole-exome data from Stransky et al . [4] revealed the occurrence of CTNNA2 mutations in three HNSCC patients. In this report, two of the three tumours originated from the larynx, whereas the remaining tumour was from the closely related and anatomically contiguous hypopharynx, providing further support to the results presented herein. Mutations in CTNNA3 were not identified in the study by Stransky et al . [4] , although this is probably because of the low number of larynx tumours examined ( n =15). This result suggests that tumours from the diverse anatomical locations constituting HNSCC may each be driven through mutation of distinct sets of genes and have important implications for patient stratification to try to improve prognostic and therapeutic approaches. In support of this, recently identified mutations of the TERT promoter in HSNCC displayed clear anatomical selectivity in oral cavity tumours, with 11 of 12 cancers with TERT promoter mutations originating from the oral tongue, despite the fact that only 23 of the total 70 HSNCC tumours were of oral tongue origin [23] . In further support of our findings, analysis of the COSMIC, cbioportal and Cancer Cell Line Encyclopedia databases [13] , [15] , [16] has revealed the annotation of many CTNNA2 and CTNNA3 mutations in a spectrum of different malignancies and tumour cell lines. These genomic data reinforce that α-catenin mutations are driver events in numerous cancer types and emphasize the need for their functional validation. The lack of any obvious primary or structural clustering in the mutations affecting CTNNA2 and CTNNA3 , and the fact that a number of them are predicted to cause premature stop codons in the encoded proteins, suggests that these mutations might prompt a loss of function in these catenins. To delve into this hypothesis, we first tested whether silencing or overexpression of these genes prompts HNSCC cells to display any cancer-related phenotype. These experiments revealed an increase in the migration and invasion capacities of cells from which these catenins had been ablated. Although the E-cadherin-α-catenin system is assumed to regulate cell–cell contacts, our result is consistent with recent reports that link E-cadherin with integrin-mediated cell–matrix adhesion in the context of tumour progression [24] . Notably, we also observed the opposite phenotype (for example, a decrease in migration and invasion capacities) in cells overexpressing any of these genes. This observation allowed us to directly test the functional consequences of the described mutations. Thus, further experiments showed that overexpression of recombinant CTNNA2 and CTNNA3 proteins harbouring several of the laryngeal carcinoma mutations cannot replicate the functional consequences of the overexpression of their wild-type counterparts. Further, the overexpression of some of these mutants seems to mimic the corresponding ablation-associated phenotype, despite the presence of the wild-type protein in those cells. This observation is consistent with a putative dominant-negative effect for these mutations. Taken together, these experiments suggest that CTNNA2 and CTNNA3 are tumour suppressor genes, and mutations in these genes in larynx cancer patients cause loss of function in both α-catenin proteins, which leads to increased migration and invasion capabilities. We then asked whether the functional changes found in these experiments could be attributed to the known role of both α-catenins as cell–cell adhesion proteins linking β-catenin to the cytoskeleton. Failure to fulfil this role might lead to deregulated release of β-catenin to the nucleus, the consequences of which are consistent with the observed phenotype. We first examined the phosphorylation status of β-catenin, which is altered in many types of cancer [16] , [17] . Interestingly, we found increased phosphorylation levels at a Ser residue implicated in the translocation of β-catenin from cell–cell contacts into the nucleus, in CTNNA2- and CTNNA3-silenced SCC-2 cells [21] . Nuclear translocation of β-catenin activates the transcription of TCF/LEF-1 family factors [22] , and, accordingly, TCF/LEF-1 luciferase reporter assays revealed a significant increase of TCF/LEF-1 transcriptional activity when CTNNA2 and CTNNA3 were ablated. Similar to the previous functional assays, overexpression of wild-type CTNNA2 and CTNNA3 also led to a measurable phenotype, with decreased β-catenin phosphorylation and TCF/LEF-1 transcriptional activity. As expected, overexpression of CTNNA2 and CTNNA3 mutants failed to replicate this wild-type phenotype, reinforcing the proposal that the described mutations impair the biological role of both α-catenins. These results suggest that acquisition of mutations in these α-catenins may inactivate a transcriptional network of genes that inhibit tumour invasion and progression [24] , [25] , [26] . Finally, our clinical data support an important role of CTNNA2 and CTNNA3 mutations on the natural history of patients with laryngeal carcinoma and are associated with worse clinical prognosis. In summary, this work has identified CTNNA2 and CTNNA3 as novel cell–cell adhesion genes frequently mutated in larynx cancer. Functional and clinical studies strongly suggest that both genes may act as tumour suppressors, which is consistent with the growing idea that the vast majority of HNSCC tumours harbour many inactivating mutations. Therefore, these α-catenins and their associated pathways offer new candidate targets for the development of strategies that may contribute to the future treatment of laryngeal carcinomas. DNA isolation from human specimens We obtained surgically resected tumour samples and matched blood samples from each patient with laryngeal carcinoma ( Table 1 ). All but one were men, all strong smokers and 62 (83%) heavy drinkers. Median age was 63 years (44–90). None of the patients received chemotherapy or radiotherapy before the surgical treatment. All the patients were treated surgically and 24 (32%) received adjuvant radiotherapy. Forty-nine (65%) were alive at last follow-up (median follow-up 40 months (0–192). The pathological stage distribution in our cohort is representative of what it is expected in this tumour (9 stage I, 17 stage II, 18 stage III and 31 stage IV). None had distant metastases at the moment of diagnosis. To obtain tumour genomic DNA, ~10 mg of fresh frozen tumour tissue were lysed in 360 μl of ATL buffer supplemented with 40 μl of proteinase K for 2–16 h. After complete macroscopic digestion, the lysate was mixed with 400 μl of AL buffer to homogenization, and then 400 μl of 100% ethanol were added, followed by thorough vortexing for 15 s and 5 min incubation at room temperature. Genomic DNA was then precipitated by 10 min centrifugation at 4 °C and 20,000 g , washed with 70% ethanol, air-dried and resuspended in 50–100 μl of AE buffer. ATL, AL, proteinase K and AE buffer were from Qiagen. Germline genomic DNA was obtained from blood samples using the Flexigene kit (Qiagen), according to manufacturer’s instructions. The experiments were conducted in accordance with the Hospital Universitario Central de Asturias Ethics Committee, and written informed consent was obtained from each individual providing biological samples. Exome enrichment Three micrograms of genomic DNA from each sample were sheared and used for the construction of a paired-end sequencing library as previously described in the paired-end sequencing sample preparation protocol provided by Illumina [27] . Enrichment of exonic sequences was then performed for each library using the Sure Select Human All Exon Kit 50 Mb (Agilent Technologies) following the manufacturer’s instructions. Exon-enriched DNA was pulled down by magnetic beads coated with streptavidin (Invitrogen), and was followed by washing, elution and 18 additional cycles of amplification of the captured library. Exon enrichment was validated by real-time PCR in a 7300 Real-Time PCR System (Applied Biosystems) using a set of two pairs of primers to amplify exons and one pair to amplify an intron. Enriched libraries were sequenced using two lanes of an Illumina GAIIx sequencer. Read mapping and processing For exome sequencing, reads from each library were mapped to the human reference genome (GRCh37) using Burrows-Wheeler Aligner [28] with the sampe option, and a BAM file was generated using SAMtools [29] . Reads from the same paired-end libraries were merged and optical or PCR duplicates were removed using Picard ( http://www.picard.sourceforge.net/index.shtml ). Statistics about the number of mapped reads and depth of coverage for each sample are shown in Supplementary Table S1 . For the identification of somatic substitutions, we used the Sidrón algorithm, which has been previously described [8] . The frequencies of machine error were estimated by examining 3 × 10 5 likely homozygous positions (coverage higher than 15, fraction of non-reference bases lower than 0.1). Because of the contamination of tumour samples with normal tissue, the cutoff S -values were lowered to 11 for positions with coverage higher than 20. The validation rate of the somatic mutations detected by Sidrón was higher than 90% as assessed by the Sanger sequencing ( Supplementary Data 5 ). Somatic mutation identification in pooled samples To discover recurrent somatic mutations in the validation series, we performed a screening in a set of 86 additional laryngeal carcinoma cases ( Supplementary Data 3 ) using a combination of pooled samples, PCR amplification and high-throughput sequencing. We used a modified method for the analysis of pooled samples [30] . Briefly, we amplified each selected exon from two pools containing equal amounts of tumour and normal DNA, respectively, from the patients. The primers used in this step are described in Supplementary Data 6 . To obtain sufficient coverage, we mixed equal amounts of the resulting 466 amplicons in four pools for each sample. Each pool was sequenced in one lane of an Illumina GAIIx sequencer for an average coverage of about 10 5 over 225,698 bases. Mutation validation To deconvolute the sequencing data generated by SMIPS, we analysed each tumour DNA from the validation set by using SNaPShot (Life Technnologies) according to the manufacturer’s instructions. We performed two separate SNaPShot reactions per tumour DNA, one for CTNNA2 and one for CTNNA3 , using the primers shown in Supplementary Table S2 . The presence of the corresponding mutation identified by SNaPShot was verified by the Sanger sequencing using a 3130XL Genetic Analyser and the primers described in Supplementary Data 6 . Cells and cell culture conditions Human HNSCC cell lines SCC-2 and SCC-40, kindly provided by Dr R. Grenman (Turku University, Finland), were cultured in DMEM (Invitrogen) supplemented with 10% fetal bovine serum, 2% HEPES, 1% non-essential amino acids and 1% penicillin-streptomycin-glutamine. Sanger sequencing experiments showed that these cell lines have no deleterious mutations in CTNNA2 or CTNNA3 . For overexpression experiments, cells at 80% confluence were transfected using Lipofectamine 2000 (Invitrogen) with the full-length human cDNA of CTNNA2 and/or CTNNA3 (Origene, RC208731 and RC226241, respectively). For knockdown experiments, cells were transduced with a set of four retroviral short-hairpin RNA vectors based on the pLKO.1 vector and designed to specifically target human CTNNA2 and/or CTNNA3 transcripts (Origene, TG313667 and TG313666, respectively). HEK-293T cells were used for virus packaging. CTNNA2 and CTNNA3 mutant DNAs were created using a Stratagene QuikChange II Site-Directed Mutagenesis kit (Agilent Technologies). Transfected clones were selected during 15 days with 400 μg ml −1 of G418 for overexpressing clones and 1.1 μg ml −1 puromycin for silencing clones. All cell lines were analysed by western blot to confirm overexpression or silencing of the selected genes. Cell adhesion assays The adhesion capacity of different cell pools was analysed with the ECM Cell Adhesion Array kit (Colorimetric; EMD Biosciences, ECM540 96 wells) following the manufacturer’s instructions. Briefly, 6 × 10 5 HNSCC cells were incubated in the ECM Array during 3 h. After cell lysis, the absorbance was measured at 485 nm using a Synergy H4 Hybrid reader. All data are the mean of three independent experiments. Time-lapse migration assays For cell migration assays, Ibidi-uncoated μ-Dishes (Ibidi 81151) were coated with laminin (15 μg ml −1 ; Sigma L2020) for 2 h at 37 °C. HNSCC cells (6 × 10 5 ) were seeded 6 h before performing the experiment on coated dishes with culture inserts (Ibidi 80209) until complete adhesion. Inserts were removed defining a cell-free gap of around 500 μm, and cells were overlayed with 2 ml of culture media. Cell migration was time-lapse recorded in a Zeiss Axiovert 200 microscope during 10 h for SCC-2 cells and 16 h for SCC-40 cells, with an XL-multi S1 incubator and using Axiovision software. Migration areas at different time points were calculated using ImageJ. In vitro invasion assays The in vitro invasion potential of HNSCC cells was evaluated using Matrigel-coated invasion chambers with an 8-μm pore size (BD Biosciences). For each experiment, 2.5 × 10 5 cells per well were allowed to migrate for 27 h for SCC-2 cells and 40 h for SCC-40 cells through the Matrigel-coated membranes using 3% fetal bovine serum as a chemoattractant. Cells that reached the lower surface of the membrane were stained. The total number of cells in the lower chamber was determined by visible light microscopy (× 4 magnification). Luciferase reporter gene assays To measure the transcriptional activity of the β-catenin/Wnt signalling pathway, HNSCC cells were transfected with the indicated vectors and seeded in 24-well plates at 1 × 10 5 cells per well. After 24 h, 0.6 μg of TCF/LEF-1 reporter (pTOP-FLASH) or control vector (pFOP-FLASH) were transiently co-transfected with 0.06 μg of TLRK vector and 0.2 μg of each DNA construct (short-hairpin RNAs, full-length wild-type and mutated cDNAs, respectively, for both CTNNA2 and CTNNA3 ) following the standard Lipofectamine 2000 protocol (Invitrogen). Cells were incubated for 24 h, and then 10 μl out of the 100 μl cell extract were used for measuring luciferase activity using the Dual Luciferase Reporter Assay System kit (Promega). Western blot Samples were subjected to SDS-PAGE and transferred to polyvinylidene difluoride (0.45 μm pore size) membranes (Millipore). Blots were blocked with 5% non-fat dry milk in TBS-T buffer (20 mM Tris-HCl pH 7.4, 150 mM NaCl and 0.05% Tween-20) for 1 h at room temperature and incubated overnight at 4 °C with 5% BSA in TBS-T with either 0.2 μg ml −1 anti-CTNNA2 (TA300943, Origene) or 0.2 μg ml −1 anti-CTNNA3 (13974-1-AP, Proteintech Europe) and 1:1000 anti α-actin (A5441, Sigma). To evaluate the phosphorylation status of β-catenin, we used β-catenin Antibody Sampler Kit (2951S, Cell Signaling). Finally, the blots were incubated for 1 h at room temperature in 2.5% non-fat dry milk in TBS-T buffer with 10 ng ml −1 of goat anti-mouse (115-035-062, Jackson ImmunoResearch) and donkey anti-rabbit (NA934V, GE Healthcare). Then, blots were washed with TBS-T and developed with Immobilon Western chemiluminescent horseradish peroxide substrate (Millipore). Chemiluminescent images were taken with a Fujifilm LAS3000 mini apparatus. Statistical analysis The SPSS Statistics 17.0 (SPSS Inc) package was employed to correlate clinical and biological variables by means of Fisher’s test or non-parametric test when necessary. Survival curves were analysed according to the Kaplan and Meier method and compared using the log-rank test. All statistical tests were two-sided and the level of statistical significance was 0.05. Accession codes: The sequencing data have been deposited in the Sequence Read Archive (SRA), under accession code PRJEB1136 . How to cite this article: Fanjul-Fernández, M. et al . Cell–cell adhesion genes CTNNA2 and CTNNA3 are tumour suppressors frequently mutated in laryngeal carcinomas. Nat. Commun. 4:2531 doi: 10.1038/ncomms3531 (2013).